T-bet and GATA3 orchestrate Th1 and Th2 differentiation through lineage-specific targeting of distal regulatory elements T-bet and GATA3 regulate the CD4+ T cell Th1/Th2 cell fate decision but little is known about the interplay between these factors outside of the murine Ifng and Il4 / Il5 / Il13 loci. Here we show that T-bet and GATA3 bind to multiple distal sites at immune regulatory genes in human effector T cells. These sites display markers of functional elements, act as enhancers in reporter assays and are associated with a requirement for T-bet and GATA3. Furthermore, we demonstrate that both factors bind distal sites at Tbx21 and that T-bet directly activates its own expression. We also show that in Th1 cells, GATA3 is distributed away from Th2 genes, instead occupying T-bet binding sites at Th1 genes, and that T-bet is sufficient to induce GATA3 binding at these sites. We propose these aspects of T-bet and GATA3 function are important for Th1/Th2 differentiation and for understanding transcription factor interactions in other T cell lineage decisions. CD4+ helper T cells respond to antigen and cytokine cues by differentiating into one of a number of specialized effector types, allowing the immune system to tailor its response to different pathogens. Failure to mount an appropriately polarized response increases the severity of infection and can induce autoimmune or allergic disorders [1] . Differentiation of CD4+ T cells into Th1 and Th2 effector cells is controlled by the transcription factors T-bet and GATA3, respectively. T-bet overexpression causes differentiation into the Th1 lineage whereas loss of T-bet induces default commitment to Th2 and Th17 lineages, resulting in impaired Th1 immunity and spontaneous asthma [2] , [3] , [4] , [5] . In contrast, deletion of Gata3 prevents differentiation into the Th2 lineage and overexpression in Th1 cells switches their polarity to a Th2 phenotype [6] , [7] . Our understanding of how T-bet and GATA3 function to regulate the Th1/Th2 cell fate decision mostly stems from the murine Ifng and Il4/Il5/Il13 loci, that encode the key Th1 and Th2 cytokines, respectively. Lineage-specific expression of these genes is dependent on a series of distal regulatory elements that act together to form domains segregated from surrounding chromatin [8] , [9] , [10] . These regulatory elements have been characterized by sequence conservation and DNaseI hypersensitivity and a number of them exhibit enhancer or insulator activity. During Th1 differentiation, T-bet directly binds to regulatory elements at the Ifng locus, leading to changes in histone modification and Ifng transcription [10] , [11] , [12] , [13] , [14] , [15] , [16] . T-bet also binds with the insulator/boundary element binding protein CTCF and the cohesin complex to conserved distal elements flanking the Ifng locus, forming intra-chromosomal loops between these elements and the Ifng gene [17] , [18] . GATA3 functions in a similar manner to activate expression of the Th2 cytokine locus, binding to multiple sites proximal and distal to Il4 , Il5 and Il13 ( [11] , [19] , [20] , [21] , [22] , [23] , [24] ). As for the Ifng locus, these distal elements are brought into proximity with promoter regions by intra-chromosomal looping [21] , [25] . T-bet and Gata3 also act through distal elements to repress the expression of Ifng and Il4 in the alternate lineage. In Th1 cells, T-bet binds to the Il4 promoter and a silencer element downstream [8] , [11] , [12] , [26] . In Th2 cells, Gata3 binding at the Ifng locus results in recruitment of polycomb repressive complex-2 (ref. 27 ). The antagonistic nature of T-bet and GATA3 is also reflected by their direct association and T-bet-mediated repression of GATA3 binding to Il5 promoter DNA [28] . Rather than being solely expressed in their specific lineage, T-bet and GATA3 are co-expressed in human Th1 cells polarized in vitro [11] , [29] , [30] , [31] and in mouse T cells after infection in vivo with lymphocytic choriomeningitis virus [32] . The co-expression of master regulator transcription factors may provide a mechanism for the functional plasticity that has been observed between T-cell effector sub-types [31] , [33] , [34] . Knowledge of the relationship between master regulator binding sites is therefore required to understand how CD4+ differentiation is controlled. However, although Th1 and Th2 cells exhibit a range of functional differences reflected by distinct programs of gene expression [1] , little is known about the relationship between T-bet and GATA3 binding outside of the Ifng and Il4/5/13 loci. To address this, and to maximize the utility of the data for our understanding human immunology, we sought to identify T-bet and GATA3 binding sites in primary human Th1 and Th2 cells by chromatin immunoprecipitation (ChIP) coupled with massively parallel sequencing (ChIP-Seq). Complemented by functional assays, this approach demonstrates how interplay between T-bet and GATA3 determines appropriate lineage differentiation. T-bet and GATA3 binding at IFNG and IL4/5/13 loci To identify T-bet and GATA3 binding sites across the human genome, we differentiated Th1 and Th2 cells in vitro from naive precursors [11] , performed ChIP for T-bet and GATA3, and generated libraries from ChIP and control input samples for Illumina sequencing. GATA3 ChIP-Seq was performed in both Th1 and Th2 cells because, unlike T-bet, it is expressed in both lineages in human ( Supplementary Fig. S1 ) [11] , [29] , [30] , [31] . We first examined T-bet and GATA3 binding at the IFNG and IL4/5/13 loci. At IFNG , we found that T-bet bound to the promoter and at both known and novel distal sites ( Fig. 1a ). The T-bet binding sites at −4, −16.2, −30.3, −44/−41.5, +22/+23.4, +39.8/+41.8 and +78.9 kb are at positions orthologous to the murine enhancers CNS−6, CNS−22, CNS−34, CNS−55, CNS+18–20, CNS+29 and CNS+46, respectively. Consistent with this, these sites are often coincident with DNaseI hypersensitive sites (DHS) and histone H3 monomethylated at lysine 4 (H3K4me1), a marker of enhancers poised to be activated upon differentiation [35] . Similarly, the T-bet binding sites at −63.5 and +119 kb correspond to previously identified CTCF-bound insulator/boundary elements [17] , [18] ( Fig. 1a ). Novel T-bet binding sites at −100, −81.4, −21.5, +147.6 and +170.2 kb overlap DHS sites and the −81.4 and −22 kb sites are also associated with H3K4me1, suggesting they also represent enhancer regions. 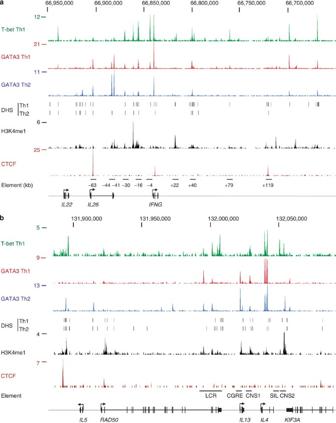Figure 1: T-bet and GATA3 binding sites at human Th1 and Th2 cytokine loci. (a) T-bet and GATA3 binding at theIFNGlocus (region shown chr12:66,650,000–66,950,000 (hg18) in reverse orientation). The number of sequencing reads from T-bet and GATA3 ChIP-enriched DNA are plotted per million background-subtracted total reads and aligned with the human genome. DHS sites in Th1 and Th2 cells are marked by dashes and sites of H3K4me1 and CTCF occupancy in resting T cells are shown below as reads per million. The positions of orthologous murine regulatory elements are indicated by the bars underneath and labelled with the approximate distance of the associated T-bet peak to theIFNGTSS. Gene structures are marked at the bottom of the figure and the start and direction of transcription with arrows. (b) Asa, except for theIL4/5/13locus (region shown chr5:131,880,000–132,090,000). Murine regulatory elements are marked; LCR, locus control region; CGRE, CG-rich element; CNS, conserved non-coding sequence; SIL, silencer. Figure 1: T-bet and GATA3 binding sites at human Th1 and Th2 cytokine loci. ( a ) T-bet and GATA3 binding at the IFNG locus (region shown chr12:66,650,000–66,950,000 (hg18) in reverse orientation). The number of sequencing reads from T-bet and GATA3 ChIP-enriched DNA are plotted per million background-subtracted total reads and aligned with the human genome. DHS sites in Th1 and Th2 cells are marked by dashes and sites of H3K4me1 and CTCF occupancy in resting T cells are shown below as reads per million. The positions of orthologous murine regulatory elements are indicated by the bars underneath and labelled with the approximate distance of the associated T-bet peak to the IFNG TSS. Gene structures are marked at the bottom of the figure and the start and direction of transcription with arrows. ( b ) As a , except for the IL4/5/13 locus (region shown chr5:131,880,000–132,090,000). Murine regulatory elements are marked; LCR, locus control region; CGRE, CG-rich element; CNS, conserved non-coding sequence; SIL, silencer. Full size image In addition to T-bet binding, we found that in Th1 cells GATA3 was also bound to each of the sites, except for those at +22, +23.4, +117 and +119 kb ( Fig. 1a ). GATA3 also showed a similar binding pattern in Th2 cells, although somewhat reduced, with binding at the −100, −4, +78.9 and +147.8 kb sites no longer detectable. The peaks of T-bet and GATA3 binding at these elements were coincident, indicating that the two factors bind to the same or closely spaced sites. These binding characteristics were repeated at the IL4/5/13 locus ( Fig. 1b ). We identified known GATA3 binding sites at the Th2 LCR, CGRE upstream of IL13 and CNS2 and, in addition, sites upstream and downstream of IL5 , elsewhere within RAD50 and at CNS1 between IL13 and IL4 . In Th1 cells, a number of the GATA3 binding sites were lost and T-bet was bound to the IL5 upstream element, the LCR, CNS1, the IL4 promoter, CNS2 and the HSIV site at the IL4 silencer. As we found for IFNG , T-bet and GATA3 binding sites were coincident at IL4/5/13 and were also often positioned at DHS and sites of H3K4me1. These results show that ChIP-Seq detects both known and novel T-bet and GATA3 binding sites at the signature Th1 and Th2 cytokine loci. T-bet and GATA3 binding at immune regulator genes We next expanded our analysis to the rest of the human genome and identified T-bet and GATA3 binding sites from statistically significant clusters of sequence reads [36] . In total, we identified 15,175 T-bet binding sites and 14,569 GATA3 binding sites in Th1 cells and 13,303 GATA3 binding sites in Th2 cells. Analysis of overrepresented sequence motifs identified a T-box binding motif enriched at sites of T-bet binding in Th1 cells and a GATA motif enriched at GATA3 binding sites in Th2 cells ( Fig. 2a ). To further assess data quality, we performed ChIP-Seq for T-bet in Th1 cells cultured from wild-type or T-bet −/− mice. We found that only 0.6% of T-bet binding sites identified in the wild-type cells were also called in the T-bet −/− cells ( Supplementary Fig. S2 ), providing further confidence in the data. 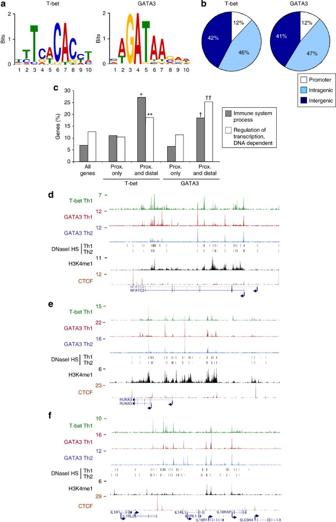Figure 2: Extensive T-bet and GATA3 binding at immune regulator genes. (a) T-bet and GATA3 binding motifs significantly enriched at the sites of T-bet and GATA3 (Th2) binding (P=2.7 × 10–65and 3.5 × 10–139, respectively,n=300). (b) Proportion of T-bet and GATA3 (Th2) binding sites that occur proximal (within 2 kb) to gene transcription start sites, within genes or between genes. (c) Percentage of genes with the enriched Gene Ontology annotations. Genes are divided into All genes, genes bound at proximal sites (<2 kb from TSS) only and genes bound at proximal and >4 distal sites. *P-value with Benjamini correction=10–10, **P=8 × 10–4, †P=4 × 10–4, ††P=5 × 10–4(n=119). (d) T-bet and GATA3 binding aroundNFATC2(region shown chr20:49,386,000–49,646,000). Details as forFig. 1a. (e) Asd, except forRUNX3(chr1:25,060,000–25,340,000). (f) Asd, except across a genomic region encodingIL1R1,IL1RL2,IL1RL1,IL18R1andIL18RAP(chr2:102,110,000–102,520,000). prox., proximal. Figure 2: Extensive T-bet and GATA3 binding at immune regulator genes. ( a ) T-bet and GATA3 binding motifs significantly enriched at the sites of T-bet and GATA3 (Th2) binding ( P =2.7 × 10 –65 and 3.5 × 10 –139 , respectively, n =300). ( b ) Proportion of T-bet and GATA3 (Th2) binding sites that occur proximal (within 2 kb) to gene transcription start sites, within genes or between genes. ( c ) Percentage of genes with the enriched Gene Ontology annotations. Genes are divided into All genes, genes bound at proximal sites (<2 kb from TSS) only and genes bound at proximal and >4 distal sites. * P -value with Benjamini correction=10 –10 , ** P =8 × 10 –4 , † P =4 × 10 –4 , †† P =5 × 10 –4 ( n =119). ( d ) T-bet and GATA3 binding around NFATC2 (region shown chr20:49,386,000–49,646,000). Details as for Fig. 1a . ( e ) As d , except for RUNX3 (chr1:25,060,000–25,340,000). ( f ) As d , except across a genomic region encoding IL1R1 , IL1RL2 , IL1RL1 , IL18R1 and IL18RAP (chr2:102,110,000–102,520,000). prox., proximal. Full size image We next assessed the location of T-bet and GATA3 binding sites across the human genome ( Supplementary Dataset 1 ). In total, we found that 88% of T-bet and GATA3 binding sites were distal (>2 kb) to known gene promoters ( Fig. 2b ). Visual inspection revealed that a number of genes exhibited extensive domains of T-bet and GATA3 binding across the locus, similar to that pattern observed at IL4/5/13 and IFNG . Across the genome, we found that 316 genes were associated with five or more distinct T-bet binding sites in Th1 cells and 295 with five or more GATA3 binding sites in Th2 cells. We asked whether any specific classes of gene were associated with these extensive patterns of T-bet and GATA3 binding. Gene Ontology revealed that genes bound by T-bet or GATA3 at proximal and multiple distal sites exhibited a significant enrichment for functions in the immune response and in transcriptional regulation ( Fig. 2c ). Genes bound by T-bet and GATA3 only at the promoter did not exhibit enrichment of these functional categories. Immune regulatory genes exhibiting concentrations of distal T-bet and GATA3 binding sites included a number with known functions in Th1 or Th2 cells, such as BATF , BCL6 , CXCR3 , ETS1 , GFI1 , HOPX , IL4R , IL2RA , IRF1 , IKZF1 ( Ikaros ), MAF , NFATC2 , PRDM1 ( Blimp1 ), RBPJ , RUNX1 , RUNX3 , STAT1 , STAT4 and STAT5 ( Fig. 2d and Supplementary Fig. S3 ). Furthermore, similar to the IL4/5/13 locus, we identified clusters of cytokine or receptor genes with extensive T-bet and GATA3 binding, for example, IL1R1/IL1RL2/IL1RL1(IL33R)/IL18R1/IL18RAP ( Fig. 2f ) and CCR9/CXCR6/XCR1/CCR1/CCR3/CCR2/CCR5/CCRL2 ( Supplementary Fig. S3 ). These results reveal that a set of key immune regulatory genes exhibit broad domains of T-bet and GATA3 binding that may be important for specific patterns of expression during T-cell differentiation. Distal elements display markers of enhancer and insulators The distal sites bound by T-bet and GATA3 at IFNG and IL4/5/13 occur at the regions of high sequence conservation and display an open chromatin confirmation, characteristic of functional elements. We therefore asked whether T-bet and GATA3 binding sites surrounding other genes shared these features. We found that distal T-bet and GATA3 binding sites were frequently located at sequences with high conservation scores (30% and 25% were classified as most conserved, respectively, compared with an expected frequency of 9%) ( Fig. 3a ) and coincided with DHS, indicative of an open chromatin conformation ( Fig. 3b ). Next, comparing sites of T-bet and GATA3 binding with the enhancer mark H3K4me1 and the boundary element factor CTCF, we found enrichment for both H3K4me1 and CTCF at distal T-bet and GATA3 binding elements ( Fig. 3c ). The coincidence of T-bet and GATA3 binding sites with DHS, H3K4me1 and CTCF can also be observed at individual loci ( Fig. 2 and Supplementary Fig. S3 ). We conclude that distal T-bet and GATA3 binding sites display markers of regulatory elements across the genome. 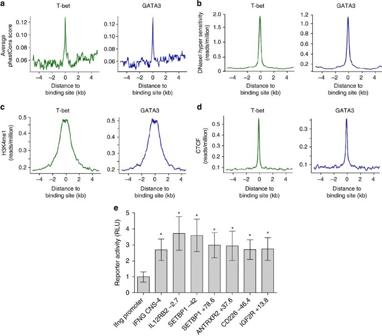Figure 3: Markers of enhancer and insulator elements at distal T-bet and GATA3 binding sites. (a) Average sequence conservation between 28 sequenced vertebrate genomes (yaxis, phastCons score) plotted against the genomic distance from a T-bet (green, left) or GATA3 (blue, right) binding site (xaxis). (b) Average number of sequence reads measuring the location of DHS sites (yaxis) plotted against the genomic distance from T-bet and GATA3 binding sites as before. (c) Average number of sequence reads from H3K4me1 ChIP DNA from resting T cells. (d) Average number of sequence reads from CTCF ChIP DNA from resting T cells. (e) Luciferase activity (firefly/renilla relative toIfngpromoter, mean and s.d., three independent transfections, performed in duplicate) in human Th0 cells transfected withIfngpromoter-driven luciferase reporter constructs with or without the named distal elements inserted upstream. *Significant increase in luciferase activity atP<0.05 (one-sidedT-test). The elements are IFNG −4 kb (P=0.0168), IL12RB2 −2.7 kb (chr1:67,542,131–67,542,929,P=0.0127), CD226 −46.4 kb (chr18:65,728,245–65,728,831,P=0.0131), ANTXR2 −37.6 kb (chr4:81,175,402–81,175,943,P=0.0254), IGF2R +13.8 kb (chr6:160,323,919–160,324,583,P=0.0179), SETBP1 −42 kb (chr18:40,471,400–40,472,121,P=0.0133) and SETBP1 +78.6 kb (chr18:40,592,792–40,593,656,P=0.0152). RLU, relative light unit. Figure 3: Markers of enhancer and insulator elements at distal T-bet and GATA3 binding sites. ( a ) Average sequence conservation between 28 sequenced vertebrate genomes ( y axis, phastCons score) plotted against the genomic distance from a T-bet (green, left) or GATA3 (blue, right) binding site ( x axis). ( b ) Average number of sequence reads measuring the location of DHS sites ( y axis) plotted against the genomic distance from T-bet and GATA3 binding sites as before. ( c ) Average number of sequence reads from H3K4me1 ChIP DNA from resting T cells. ( d ) Average number of sequence reads from CTCF ChIP DNA from resting T cells. ( e ) Luciferase activity (firefly/renilla relative to Ifng promoter, mean and s.d., three independent transfections, performed in duplicate) in human Th0 cells transfected with Ifng promoter-driven luciferase reporter constructs with or without the named distal elements inserted upstream. *Significant increase in luciferase activity at P <0.05 (one-sided T -test). The elements are IFNG −4 kb ( P =0.0168), IL12RB2 −2.7 kb (chr1:67,542,131–67,542,929, P =0.0127), CD226 −46.4 kb (chr18:65,728,245–65,728,831, P =0.0131), ANTXR2 −37.6 kb (chr4:81,175,402–81,175,943, P =0.0254), IGF2R +13.8 kb (chr6:160,323,919–160,324,583, P =0.0179), SETBP1 −42 kb (chr18:40,471,400–40,472,121, P =0.0133) and SETBP1 +78.6 kb (chr18:40,592,792–40,593,656, P =0.0152). RLU, relative light unit. Full size image We next sought to verify that distal T-bet binding sites that overlap regions of H3K4me1 function as enhancers. We cloned the distal binding sites at IL12RB (−2.7 kb), SETBP1 (−42 kb) , SETBP1 (+78.6 kb) , ANTXR2 (−37.6 kb), CD226 (−46.4 kb) and IGF2R ( +13.8 kb ), and inserted them upstream of the basal murine Ifng promoter driving a luciferase reporter. We then transfected these constructs into activated human CD4+ T cells and measured luciferase activity ( Fig. 3e ). We found that each of these elements enhanced luciferase expression compared with the Ifng promoter alone and conclude that distal T-bet and GATA3 binding sites identified by ChIP-Seq function as regulatory elements. Distal sites are associated with lineage-specific expression The association of distal binding sites with markers of enhancer or insulator function suggested that T-bet and GATA3 regulate their gene expression through these sites. To test this, we activated purified naive CD4+ T cells, cultured them in either Th1 or Th2 polarizing conditions and identified changes in expression using microarrays. We found that ~40% of genes with both proximal and distal T-bet and GATA3 binding sites exhibited changes in expression during T-cell activation, compared with only 20% of genes bound at proximal sites alone ( Fig. 4a ). Furthermore, genes bound by T-bet or GATA3 at both proximal and distal sites were more than twice as likely to show differential expression between Th1 and Th2 lineages in both human and mouse T cells ( Fig. 4a ). This was not a statistical effect of the increasing number of binding sites ( Supplementary Fig. S4 ), and these results demonstrate that T-bet and GATA3 binding at promoter and distal sites correlate with changes in gene expression during T-cell differentiation. 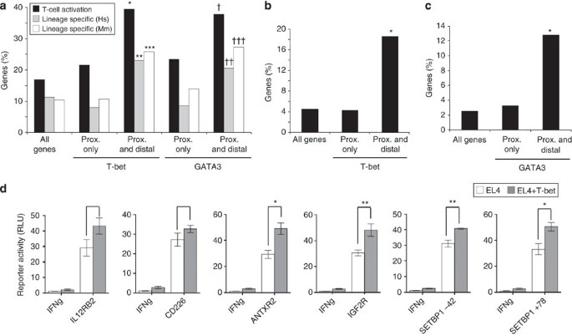Figure 4: Distal binding sites are associated with differential expression and regulation by T-bet and GATA3. (a) Percentage of genes that show changes (>2-fold) in gene expression during differentiation of naive mouse CD4+ T cells to Th1 or Th2 effector cells (black), differential gene expression (2-fold) between human Th1 and Th2 cells (grey) or between mouse Th1 and Th2 cells (white). Genes are divided into all genes, genes bound by T-bet or GATA3 proximally and genes bound by T-bet or GATA3 proximally and distally (>2 sites). *Significant association between binding and expression atP<10–16(n=213), **P=8 × 10–8(n=243), ***P=10–11(n=237), †P=10–11(n=180), ††P=6 × 10–5(n=204), †††P=2 × 10–11(n=198). (b) Percentage of genes that exhibit differential gene expression (>2-fold) in T cells from T-bet-deficient mice cultured under Th1 conditions compared with cells from wild-type mice. Genes are divided into the same sets as A. *P<10–16(n=237). (c) Percentage of genes that exhibit differential gene expression (>2-fold) in Gata3-deficient T cells cultured under Th2 conditions compared with cells from wild-type mice. *P=2 × 10–10(n=180). (d) Luciferase activity (mean and s.e., three independent experiments) in EL4 cells and EL4 cells stably expressing T-bet transfected withIfngpromoter-driven luciferase reporter constructs with or without the named distal elements inserted upstream (details as forFig. 3e). *P<0.02, **P<0.01.P-values are 0.064, 0.11, 0.011, 0.008, 0.006, 0.016, respectively (EL4 T-bet versus EL4, one-sidedT-test). prox., proximal. RLU, relative light unit. Figure 4: Distal binding sites are associated with differential expression and regulation by T-bet and GATA3. ( a ) Percentage of genes that show changes (>2-fold) in gene expression during differentiation of naive mouse CD4+ T cells to Th1 or Th2 effector cells (black), differential gene expression (2-fold) between human Th1 and Th2 cells (grey) or between mouse Th1 and Th2 cells (white). Genes are divided into all genes, genes bound by T-bet or GATA3 proximally and genes bound by T-bet or GATA3 proximally and distally (>2 sites). *Significant association between binding and expression at P <10 –16 ( n =213), ** P =8 × 10 –8 ( n =243), *** P =10 –11 ( n =237), † P =10 –11 ( n =180), †† P =6 × 10 –5 ( n =204), ††† P =2 × 10 –11 ( n =198). ( b ) Percentage of genes that exhibit differential gene expression (>2-fold) in T cells from T-bet-deficient mice cultured under Th1 conditions compared with cells from wild-type mice. Genes are divided into the same sets as A. * P <10 –16 ( n =237). ( c ) Percentage of genes that exhibit differential gene expression (>2-fold) in Gata3-deficient T cells cultured under Th2 conditions compared with cells from wild-type mice. * P =2 × 10 –10 ( n =180). ( d ) Luciferase activity (mean and s.e., three independent experiments) in EL4 cells and EL4 cells stably expressing T-bet transfected with Ifng promoter-driven luciferase reporter constructs with or without the named distal elements inserted upstream (details as for Fig. 3e ). * P <0.02, ** P <0.01. P -values are 0.064, 0.11, 0.011, 0.008, 0.006, 0.016, respectively (EL4 T-bet versus EL4, one-sided T -test). prox., proximal. RLU, relative light unit. Full size image To confirm a functional role for T-bet and GATA3 binding to distal sites across the genome, we asked whether they were associated with a requirement for T-bet or GATA3 for gene regulation. We first compared gene expression in Th1 cells cultured from wild-type and T-bet-deficient mice ( Fig. 4b ). In total, around 4% of genes showed a requirement for T-bet for normal expression in Th1 cells. For genes bound by T-bet at proximal sites alone, we found that the frequency of gene expression changes was also ~4% showing that T-bet was not required for their regulation. In contrast, genes bound by T-bet at proximal and distal sites were four times more likely to be dependent on T-bet for their expression ( P <10 –16 , n =237). To perform this test for GATA3, we purified naive T cells from wild-type mice and from animals in which Gata3 is deleted from activated T cells [37] and differentiated these under Th2 conditions. As we discovered for T-bet, loss of Gata3 had no effect on genes that were only associated with GATA3 at proximal sites but genes also bound at distal sites were four times as likely to be dependent on Gata3 for their expression ( P =1.6 × 10 –10 , n =180). These results show that although T-bet and GATA3 can bind genes at the promoter alone, distal sites at immune regulator genes are required for both factors to effect changes in gene expression. To verify that T-bet can act through these newly identified distal binding sites, we assayed the activity of reporter gene constructs in murine EL4 cells in the presence and absence of T-bet ( Fig. 4d ). Each of these elements bound T-bet in their genomic context ( Supplementary Fig. S3 ). We found that the inclusion of these elements upstream of the Ifng promoter led to increased luciferase activity and this was further enhanced by the presence of T-bet. Together with the microarray data, these results illustrate the importance of distal elements for T-bet and GATA3-mediated control of immune regulatory genes. T-bet binds and directly activates expression of its own gene One locus at which we detected extensive distal T-bet and GATA3 binding was TBX21 , which encodes T-bet itself ( Fig. 5a ). Furthermore, consistent with previous findings [38] , these binding sites were associated with Th1-specific DHS and with H3K4me1, indicating enhancer function. To verify enhancer function, we cloned the genomic region around the −11 and +7.8 kb binding sites upstream of a luciferase reporter construct driven by the basal Ifng promoter and expressed these in human ( Fig. 5b and Supplementary Fig. S6m ) and mouse ( Fig. 5c ) Th0 and Th2 cells. We found that the Tbx21 −11 kb element resulted in Th0-specific enhancement of luciferase activity. We conclude from this that expression of T-bet could potentially be directly regulated by T-bet itself. 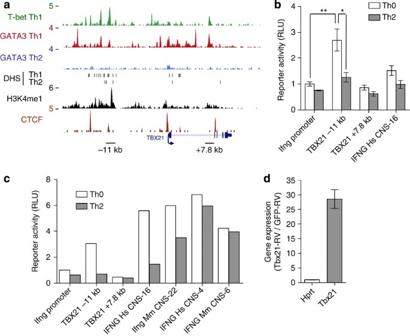Figure 5: T-bet binding and auto-activation ofTbx21. (a) T-bet and GATA3 binding at the humanTbx21locus. Details as forFig. 1. The positions of the T-bet binding elements assayed inbare indicated by dashed boxes. (b) Luciferase activity (mean and s.e., one donor, three transfections) in human Th0 (white) and Th2 (grey) cells transfected withIfngpromoter-driven luciferase reporter constructs with or without the named distal elements inserted upstream. **P=0.001, *P=0.003 (one-sidedT-test). Th1 cells were not viable after nucleofection. (c) Luciferase activity in mouse Th0 (white) and Th2 (grey) cells (n=1) transfected withIfngpromoter-driven luciferase reporter constructs with or without the named distal elements inserted upstream. (d) Expression of endogenousTbx21mRNA andHprtmRNA (mean and s.d., two independent experiments) in Ifnγ−/−CD4+ T cells transduced with T-bet-GFP retrovirus relative to cells transduced with control GFP retrovirus. RLU, relative light unit. Figure 5: T-bet binding and auto-activation of Tbx21 . ( a ) T-bet and GATA3 binding at the human Tbx21 locus. Details as for Fig. 1 . The positions of the T-bet binding elements assayed in b are indicated by dashed boxes. ( b ) Luciferase activity (mean and s.e., one donor, three transfections) in human Th0 (white) and Th2 (grey) cells transfected with Ifng promoter-driven luciferase reporter constructs with or without the named distal elements inserted upstream. ** P =0.001, * P =0.003 (one-sided T -test). Th1 cells were not viable after nucleofection. ( c ) Luciferase activity in mouse Th0 (white) and Th2 (grey) cells ( n =1) transfected with Ifng promoter-driven luciferase reporter constructs with or without the named distal elements inserted upstream. ( d ) Expression of endogenous Tbx21 mRNA and Hprt mRNA (mean and s.d., two independent experiments) in Ifnγ −/− CD4+ T cells transduced with T-bet-GFP retrovirus relative to cells transduced with control GFP retrovirus. RLU, relative light unit. Full size image To address whether T-bet is capable of directly inducing Tbx21 expression, CD4+ T cells were transduced with a retrovirus (RV) expressing T-bet and GFP, and a control RV expressing GFP alone. To rule out autocrine activation of Tbx21 expression through Ifnγ and Stat1, the experiment was performed with cells from Ifnγ −/− mice [39] . We found that expression of T-bet from the RV construct resulted in a marked increase in endogenous Tbx21 transcript levels compared with control-RV-infected cells ( Fig. 5d ). Also independently of Ifnγ, T-bet directly activated the expression of other genes to which it was bound, including those involved in T-cell trafficking ( Itgal , Icam1 ), cytotoxicity ( Faslg , Gzmb ) and inflammation ( Lta ) ( Supplementary Figs S5 and S6 ). These results demonstrate that T-bet can directly activate its own gene and other genes in an Ifnγ-independent manner, supporting the notion that T-bet acts through distal elements to directly reinforce Th1 lineage commitment. Alternative GATA3 distribution at T-bet sites in Th1 cells Visual inspection of the data indicated that many distal elements were bound by GATA3 in a lineage-specific manner. Performing a more systematic analysis across the genome, we found that around 1/4 of GATA3 sites were specific to Th1 cells (24.7%) and another 1/4 were specific to Th2 cells (23.6%) ( Fig. 6a , Supplementary Fig. S7 , Supplementary Dataset 2 ). This shows that GATA3 exhibits an alternative genomic distribution in Th1 versus Th2 cells. Given that T-bet and GATA3 often bind to the same sites, we asked whether the alternative distribution of GATA3 in Th1 cells reflected an association with T-bet binding sites. Comparison between T-bet and GATA3 revealed that around half (48.3%) of the Th1-specific GATA3 binding sites were coincident with T-bet binding elements ( Fig. 6a ). In contrast, only 5.6% of Th2-specific GATA3 binding sites were coincident with T-bet binding elements. Thus, GATA3 displays an alternate distribution at distal elements in Th1 cells that more closely resembles that of T-bet. 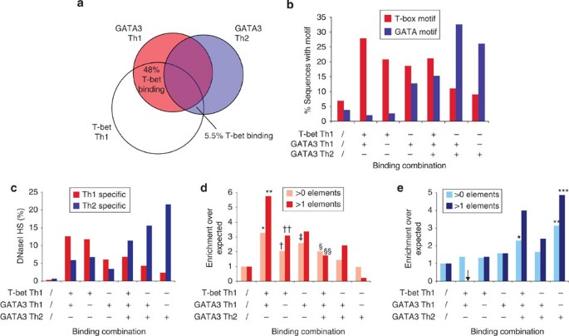Figure 6: GATA3 adopts alternate distributions in Th1 and Th2 cells. (a) Venn diagram showing the distal elements occupied by T-bet in Th1 cells, GATA3 in Th1 cells and GATA3 in Th2 cells. The percentage of elements bound by GATA3 specifically in Th1 cells or specifically in Th2 cells that are also occupied by T-bet are indicated. (b) Frequency of GATA and T-box motifs at distal sites exhibiting the six observed binding combinations of T-bet and GATA3 in Th1 and Th2 cells. The percentage of random sites that contain each motif is indicated for comparison. (c) Percentage of binding sites with each combination which are coincident with a Th1-specific (red) or a Th2-specific (blue) DHS site. The percentage of random sites that are coincident with a DHS site is indicated for comparison. (d) Fold-enrichment in the number of genes overexpressed in Th1 cells compared with Th2 cells (2-fold) for genes associated with at least one or at least two elements exhibiting each of the six different transcription factor occupancy combinations. *P=2 × 10–11(n=460), **P=3 × 10–6(n=72), †P=4 × 10–13(n=1,726), ††P=10–11(n=538), ‡P=2 × 10–6(n=436), §P=7 × 10–7(n=950), §§P=6 × 10–5(n=279). (e) As ford, except for genes overexpressed in Th2 cells compared with Th1 cells (2-fold). *P=2 × 10–11(n=950), **P=3 × 10–6(n=778), ***P=4 × 10–13(n=153). Figure 6: GATA3 adopts alternate distributions in Th1 and Th2 cells. ( a ) Venn diagram showing the distal elements occupied by T-bet in Th1 cells, GATA3 in Th1 cells and GATA3 in Th2 cells. The percentage of elements bound by GATA3 specifically in Th1 cells or specifically in Th2 cells that are also occupied by T-bet are indicated. ( b ) Frequency of GATA and T-box motifs at distal sites exhibiting the six observed binding combinations of T-bet and GATA3 in Th1 and Th2 cells. The percentage of random sites that contain each motif is indicated for comparison. ( c ) Percentage of binding sites with each combination which are coincident with a Th1-specific (red) or a Th2-specific (blue) DHS site. The percentage of random sites that are coincident with a DHS site is indicated for comparison. ( d ) Fold-enrichment in the number of genes overexpressed in Th1 cells compared with Th2 cells (2-fold) for genes associated with at least one or at least two elements exhibiting each of the six different transcription factor occupancy combinations. * P =2 × 10 –11 ( n =460), ** P =3 × 10 –6 ( n =72), † P =4 × 10 –13 ( n =1,726), †† P =10 –11 ( n =538), ‡ P =2 × 10 –6 ( n =436), § P =7 × 10 –7 ( n =950), §§ P =6 × 10 –5 ( n =279). ( e ) As for d , except for genes overexpressed in Th2 cells compared with Th1 cells (2-fold). * P =2 × 10 –11 ( n =950), ** P =3 × 10 –6 ( n =778), *** P =4 × 10 –13 ( n =153). Full size image We examined transcription factor binding motifs to determine whether there were any differences that may explain why GATA3 occupied different elements in Th2 and Th1 cells ( Fig. 6b ). As expected, we could often identify a GATA motif at sites occupied by GATA3 specifically in Th2 cells, with the T-box motif detected less frequently. In contrast, sites occupied by both T-bet in Th1 cells and GATA3 in Th2 cells exhibited T-box and GATA motifs at equal frequency. Surprisingly, at sites occupied by T-bet and GATA3 specifically in Th1 cells, only the T-box motif was present, with background occurrence of the GATA motif ( Fig. 6b ). These data support the conclusion that the Th1-specific distribution of GATA3 is not mediated through binding to its cognate GATA site but instead occurs through an association with T-bet and the T-box motif. Specific binding patterns associated with lineage specificity We next considered the functional role of the alternate GATA3 binding distribution in Th1 cells. We first sought to verify that lineage-specific binding at distal sites correlated with DHS patterns ( Fig. 6c ). As expected, we found that sites occupied specifically in Th1 cells tended to exhibit Th1-specific DNaseI hypersensitivity and sites occupied by GATA3 only in Th2 cells exhibited Th2-specific DNaseI hypersensitivity. We next sought to measure the influence of different T-bet and GATA3 binding distributions at distal sites on differential gene expression between Th1 and Th2 cells. For each pattern of transcription factor occupancy that occurred at distal sites, we calculated the frequency at which the associated gene was overexpressed in Th1 or Th2 cells compared with the frequency for all genes ( Fig. 6d ). We found that genes with a Th1-specific binding site were more likely to be overexpressed in Th1 cells but no more likely to be overexpressed in Th2 cells than expected. Genes with sites bound by T-bet and GATA3 specifically in Th1 cells exhibited the highest frequency of Th1-specific expression (up to 6-fold higher than expected P =2 × 10 –11 , n =460). In contrast, genes associated with a Th2-specific GATA3 binding site were more likely to be overexpressed in Th2 cells ( P =10 –12 , n =778) and less likely to be a Th1-specific gene than expected. The binding of GATA3 to Th1-specific sites did not alter the expression of the associated genes ( Supplementary Fig. S7c ). Rather, this alternative distribution of GATA3 away from Th2-specific to Th1-specific sites was associated with the repression of Th2-specific expression programs in Th1 cells. T-bet causes GATA3 binding at Th1-specific sites The binding of GATA3 to T-bet binding sites that lack a GATA motif in Th1 cells suggested that the redistribution of GATA3 to these sites was caused by T-bet. To test this, we generated a set of EL4 cell lines that stably expressed FLAG-T-bet or HA-Gata3 individually or together. We performed ChIP with anti-FLAG and anti-HA antibodies and quantified enrichment of mouse sequences orthologous to human distal binding sites by real-time PCR. We found that ChIP for HA-Gata3 resulted in high enrichment of the Il4 CNS2 element, consistent with our ChIP-Seq analysis that had defined this as a Th2-specific Gata3 binding site ( Fig. 7a ). In the presence of T-bet, Gata3 association with this element was reduced. We next examined T-bet and Gata3 binding at Th1-specific sites at Ifng (CNS-6) and Tbx21 (−11 kb element) ( Fig. 7b ). Both sites were bound by T-bet, confirming our ChIP-Seq data. In the absence of T-bet, Gata3 was not associated with either of these elements but when T-bet was co-expressed, Gata3 became bound. These results were recapitulated using a second set of EL4 lines ( Supplementary Fig. S8 ). We conclude from these data that T-bet is sufficient to induce Gata3 occupancy at Th1-specific sites. 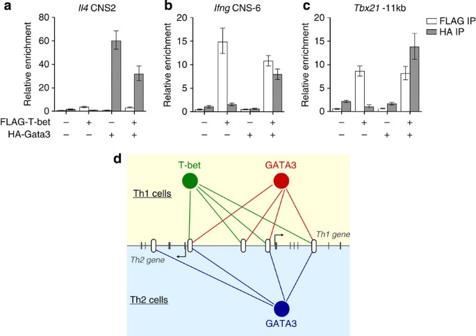Figure 7: T-bet co-expression induces GATA3 occupancy at T-bet binding sites. (a) Enrichment ofIl4CNS2 DNA (mean and s.d.,n=3) by ChIP with anti-FLAG or anti-HA antibodies relative to input DNA measured by quantitative PCR. ChIPs were performed in four stable EL4 cell lines expressing FLAG-tagged T-bet, HA-tagged Gata3, neither protein or both proteins together. Data are normalized to a control region withinDleu2that lacks T-bet and GATA3 binding sites. (b) Asa., except forIfngCNS-6. (c) Asa, except for the murine ortholog of theTbx21−11-kb element. (d) Model. T-bet and GATA3 act through distal elements to control expression of immune regulator genes. The alternate distribution of GATA3 from Th2-specific GATA sites to a set of Th1-specific T-bet binding sites is associated with a switch from Th2 to Th1-specific expression. Figure 7: T-bet co-expression induces GATA3 occupancy at T-bet binding sites. ( a ) Enrichment of Il4 CNS2 DNA (mean and s.d., n =3) by ChIP with anti-FLAG or anti-HA antibodies relative to input DNA measured by quantitative PCR. ChIPs were performed in four stable EL4 cell lines expressing FLAG-tagged T-bet, HA-tagged Gata3, neither protein or both proteins together. Data are normalized to a control region within Dleu2 that lacks T-bet and GATA3 binding sites. ( b ) As a ., except for Ifng CNS-6. ( c ) As a , except for the murine ortholog of the Tbx21 −11-kb element. ( d ) Model. T-bet and GATA3 act through distal elements to control expression of immune regulator genes. The alternate distribution of GATA3 from Th2-specific GATA sites to a set of Th1-specific T-bet binding sites is associated with a switch from Th2 to Th1-specific expression. Full size image Our understanding of how T-bet and GATA3 regulate the Th1-Th2 lineage decision mostly stems from analysis of the murine Ifng and Il4/5/13 loci. Our comparison of T-bet and GATA3 binding in human T cells has allowed us to make a number of new discoveries and delineate general principles for T-bet and GATA3 function ( Fig. 7d ). First, T-bet and GATA3 associate with distal elements across the genome and these are concentrated at a set of key immune regulatory genes. Second, these distal binding sites have the characteristics of regulatory elements and are associated with the ability of T-bet and GATA3 to exert effects on gene expression. Third, such binding sites at TBX21 allow T-bet to directly activate its own expression. Finally, in Th1 cells, GATA3 is redistributed away from distal sites at Th2 genes to T-bet binding sites at Th1 genes, and T-bet is sufficient to induce GATA3 binding at these sites. Previous studies have found that T-bet and GATA3 associate with hundreds of genes with various roles of which only a minority showed differential expression between Th1 and Th2 cells [11] , [40] , [41] . We have now been able to show that although T-bet and GATA3 do associate with the promoters of many genes, there is a specific set of immune regulators that are associated with multiple distal binding sites. These distal elements exhibit markers of enhancer or boundary element function and often stretch up and downstream of the gene or across clusters of related genes. These findings are consistent with the large cis -regulatory regions required for lineage-specific expression of Ifng and Il4/5/13 and suggest that such concentrations of T-bet and GATA3 binding sites function across the genome to define regulatory domains that govern gene expression during T cell differentiation. Our genome-wide analysis has revealed how T-bet and GATA3 binding sites are related to each other in the genome. In Th2 cells, GATA3 binds to a unique set of sites that contain a GATA motif and which are associated with Th2-specific expression. In Th1 cells, GATA3 is distributed away from these sites and instead occupies sites that are often also bound by T-bet. This sequestering of GATA3 away from Th2 genes would prevent the activation of these genes in Th1 cells. Expression of T-bet is sufficient to induce GATA3 binding at Th1-specific sites, indicating it is directly responsible for the redistribution of GATA3 in Th1 cells. Consistent with this, T-bet can interact with GATA3 and prevent its binding to the Il5 promoter [28] . The redistribution of a transcription factor by another factor has previously been identified as a strategy for the differential regulation of gene expression between two cellular states [42] and may therefore also underlie the generation of alternative transcriptional programs in T cells. The maintenance of GATA3 expression in human Th1 cells, but in an alternative distribution, may also allow for the degree of functional plasticity observed in human effector T cells [31] , [34] . It will be interesting to discover whether co-expression of other pairs of master regulators, such as T-bet and FoxP3 (refs 43 , 44 , 45 ) and Rorγt and FoxP3 (ref. 46 ), is also associated with the adoption of alternate genomic distributions. The binding of T-bet and GATA3 to distal elements at key regulators of Th1 and Th2 function places them at the root of a regulatory network that orchestrates CD4+ T-cell differentiation. This highlights how regulation of IFNG and IL4/5/13 by T-bet and GATA3 represents only one aspect of the functions of these factors in lineage specification. Providing a demonstration of the function of T-bet outside of IFNG and IL4/5/13 , we have discovered that T-bet acts at distal elements to activate its own expression. Positive feedback loops allow cell fate decisions to be regulated as a bistable switch, which convert a graduated input into a binary response [47] and such auto-activation has also been observed for GATA3 (ref. 48 ) and FoxP3 (ref. 48 ). Thus, T-bet auto-activation likely allows the cell to rapidly upregulate T-bet in response to a threshold of IL-12 signalling and then maintain T-bet expression, even when IFNγ is limiting. In summary, we have discovered that T-bet and GATA3 function through extended cis -regulatory regions to control the expression of a set of key immune regulatory genes and that T-bet acts to redistribute GATA3 to T-bet binding sites at Th1 genes. This work greatly expands our knowledge of the role of T-bet and GATA3 in T-cell differentiation and of the regulatory elements through which they act. Knowledge on this broader scale will likely be important for understanding and treating immunopathologies and will have implications for other T-cell master regulators and CD4+ effector types. Mice Wild-type BALB/c mice are from Harlan Laboratories (Indianapolis, IN, USA), T-bet−/− mice (BALB/c background) from Taconic (Ejby, Denmark) and Ifnγ−/− mice from the Jackson Laboratory [39] . ChIP-Seq Naive human CD4+ T cells were isolated and polarized as described [11] . Cells were crosslinked with formaldehyde, lysed and sonicated at 24 W for 10 × 30 s pulses using a Misonix Sonicator 3000. The resulting whole-cell extract was incubated overnight at 4 °C with Dynal Protein G beads preincubated with 10 μl of purified serum (T-bet antibody 9856 [50] ) or 10 μg of anti-GATA3 (D-16, Santa Cruz). Beads were washed and bound complexes eluted and crosslinks reversed by heating at 65 °C. IP and input DNA were then purified by treatment with RNAseA, proteinase K and phenol:chloroform extraction. Libraries were constructed from IP and input DNA by standard Illumina protocols, except that DNA in the range 150–350 bp was gel purified after PCR amplification. The library was quantified using an Agilent bioanalzer and subjected to 35-bp single-end read sequencing with an Illumina Genome Analyzer II. Data analysis Initial processing was performed with the CASAVA pipeline. Reads were aligned to the hg18 build of the human genome with ELAND and background corrected normalized tag density calculated. Significant peaks of T-bet and GATA3 binding were identified with MACS [36] . We generally used a P -value threshold of 10 –6 but varied this to identify specific combinations of T-bet and GATA3 binding. Distal binding sites (>4 kb from TSS) were assigned to the gene with the nearest TSS that was also bound proximally by T-bet or GATA3 (<2 kb from TSS). The significance of the association between transcription factor binding and change in gene expression was calculated using the hypergeometric distribution. Significant motifs were identified using MEME. Significantly enriched functional gene categories were identified using DAVID ( http://david.abcc.ncifcrf.gov/ ). DNaseI hypersensitivity data are from the University of Washington ENCODE group [18] . H3K4me1 and CTCF ChIP-Seq data are from Barski et al . [51] Gene expression microarrays Naive murine CD4+ T cells (CD4+CD25-CD62LhighCD44low) were activated and polarized in vitro for 7 days. Cells were reactivated with phorbol myristate acetate (PMA) (50 ng ml −1 ) and ionomycin (1 μg ml −1 ) for 4 h and then lysed in TRIzol (Invitrogen). Gene expression analysis was performed using Affymetrix GeneChip Mouse Gene 1.0 ST arrays (T-bet experiment) or Mouse Genome 430A 2.0 arrays (Gata3 experiment), according to the manufacturer’s instructions. Arrays images were analysed using Microarray Analysis Suite 5.0 with the default settings, and normalization was performed by robust multi-array average. For comparison to T-bet and GATA3 binding results, data for multiple transcripts were averaged for each gene. Gene expression data from human Th1 and Th2 cells were described previously [11] . Enhancer reporter assays Distal binding elements were amplified (primers in Supplementary Methods ) and cloned upstream of the murine Ifng promoter (−591 to +42 bp) in the luciferase reporter vector pGL4.13 (Promega). For assaying enhancer activity ( Fig. 3e ), naive human CD4+ cells were activated for 72 h with anti-CD3/CD28 and cultured for an additional 72 h in the presence of IL2 only. Cells were then transfected with reporter plasmid and control Renilla plasmid pRL-TK (Promega) using nucleofection (Nuclofector 4D, Lonza) and reactivated with anti-CD3/CD28 for 6 h before assaying for luciferase activity. For lineage-specific measurement of Tbx21 enhancer activity, naive mouse or human cells were initially activated for 3 days under polarizing conditions, with IL2 (Th0) or IL4 and anti-IFNγ (Th2) (Th1 cells were not viable after transfection) and then cultured for additional 72 h (mouse) or 7 days (human). Cells were then transfected and reactivated in the presence of 20 ng ml −1 IL-12 (eBioscience). To measure the effect of T-bet on enhancer activity, we generated an EL4 cell line that stably expressed T-bet under blasticidin resistance and a control cell line only expressing the selectable marker. Luciferase activities were determined using the Dual Luciferase Reporter Assay System (Promega). Retroviral expression of T-bet HEK293T cells were transfected with pMIG-T-bet and pCL-Eco (Imgenex) using polyethyleneimine and viral supernatants collected 48 h later. Naive mouse T cells from Ifng−/− mice were sorted and maintained as before. After activation for 24 h with anti-CD3 and anti-CD28, cells were transduced in the presence of 8 μg ml −1 polybrene. Cells were activated for an additional 48 h and then cultured for 3 days with IL2. Total RNA was isolated, treated with Turbo-DNaseI (Ambion), reverse transcribed with oligo-dT primers and endogenous Tbx21 mRNA measured by quantitative PCR (Applied Biosystems). Expression values were normalized to Hprt . T-bet and Gata3 co-expression FLAG-tagged T-bet was fused to the blasticidin resistance gene using a 2A sequence to obtain co-translational expression and incorporated into the pMY-IRES-GFP retroviral vector (gift from Adrian Hayday). HA-tagged Gata3 was fused to the puromycin resistance gene and incorporated into pMY-IRES-mPlum. Stable EL4 cell lines were transduced and then selected to express either GFP and mPlum, FLAG-T-bet and mPlum, HA-Gata3 and GFP or FLAG-T-bet and HA-Gata3. ChIP was performed as above, except with sonication at 30 W for 13 × 30 s pulses and with antibodies against HA (3F10, Roche) and FLAG (M2, Sigma). Enrichment of T-bet and Gata3 binding sites relative to input DNA and a control region in Dleu2 were determined by quantitative PCR (primers in Supplementary Methods ). Supplementary Information contains Supplementary Methods , two Supplemental Data files and eight Supplementary Figures . All raw and processed ChIP-Seq data are available at GEO under accession number GSE31320 . Mouse array data can be accessed at ArrayExpress under accession number E-TABM-1187 . How to cite this article: Kanhere, A. et al . T-bet and GATA3 orchestrate Th1 and Th2 differentiation through lineage-specific targeting of distal regulatory elements. Nat. Commun. 3:1268 doi: 10.1038/ncomms2260 (2012).